MYC/MIZ1-dependent gene repression inversely coordinates the circadian clock with cell cycle and proliferation The circadian clock and the cell cycle are major cellular systems that organize global physiology in temporal fashion. It seems conceivable that the potentially conflicting programs are coordinated. We show here that overexpression of MYC in U2OS cells attenuates the clock and conversely promotes cell proliferation while downregulation of MYC strengthens the clock and reduces proliferation. Inhibition of the circadian clock is crucially dependent on the formation of repressive complexes of MYC with MIZ1 and subsequent downregulation of the core clock genes BMAL1 ( ARNTL ), CLOCK and NPAS2 . We show furthermore that BMAL1 expression levels correlate inversely with MYC levels in 102 human lymphomas. Our data suggest that MYC acts as a master coordinator that inversely modulates the impact of cell cycle and circadian clock on gene expression. Many aspects of mammalian physiology and behaviour are rhythmically regulated by the circadian clock [1] . On a cellular level, the circadian clock is dependent on interconnected transcriptional/translational feedback loops. In brief, the core transcription activator complex BMAL1/CLOCK (or its homologue BMAL1/NPAS2) rhythmically activates expression of clock genes including CRYs , PERs , REV-ERBs and RORs . CRYs and PERs are inhibitors of CLOCK/BMAL, whereas REV-ERBs are repressors that control in coordination with ROR activators expression of BMAL1 , CLOCK and NPAS2 . The D-box-specific transcription factors E4BP, DBP, TEF and HLF additionally contribute to the regulation of specific clock genes [2] . Disruption or misalignment of circadian rhythms in humans has been associated with numerous pathological conditions including cancer [3] , [4] . Mice with chronic jet-lag or disrupted circadian physiology due to lesions of their suprachiasmatic nuclei exhibit accelerated growth of tumours [5] , [6] . Vice versa, cancer types correlating with impaired cell cycle and proliferation frequently exhibit aberrant expression of clock genes [7] , [8] . MYC is an oncogene, which is found to be deregulated in different cancers and, amplification of MYC often correlates with tumour aggression and poor prognosis [9] . MYC and its partner MAX are, like the circadian transcription factors BMAL1, CLOCK and, NPAS2, members of the bHLH transcription factors family, which form heterodimers that bind to so-called E-box motifs. MYC regulates transcription of up to 15% of the transcriptome including genes involved in apoptosis, cell growth and proliferation [10] , [11] . Recently, MYC has been suggested to attenuate the circadian clock by activating via circadian E-box sites transcription and expression of REV-ERBα/β, which would then repress transcription of BMAL1 (ref. 12 ). Since the DNA-binding specificity of MYC/MAX and CLOCK/BMAL1 complexes is highly similar, it seems conceivable that overexpressed MYC could constitutively activate and overexpress the E-box-dependent circadian repressor genes REV-ERBα/β , PER1/2 and CRY1/2 . Here we show, that overexpression of MYC attenuates the circadian clock of U2OS cells. Downregulation of the clock by overexpressed MYC is dependent on MYC/MIZ1 complexes, which are recruited to non-E-box sites in the promoters of BMAL1 and CLOCK . MYC/MIZ1 complexes stimulate proliferation of U2OS cells, suggesting that MYC inversely correlates the circadian clock and the cell cycle. BMAL1 and MYC share common target genes We therefore tested whether and how MYC/MAX and CLOCK/BMAL1 might regulate common circadian genes. A comparison of published chromatin immunoprecipitation sequencing (ChIP-seq) data sets of U2OS cells revealed a significant overlap between both cistromes, with 28% (574/2048) of BMAL1 binding sites overlapping with sites also bound by MYC (refs 13 , 14 ; Fig. 1a ). Such common binding sites include the core circadian clock genes REV-ERBα, PER1/2 and DBP as well as clock-controlled genes such as SCN5A ( Fig. 1b and Supplementary Fig. 1a ). However, co-transfection of HEK293 cells with MYC/MAX expressing constructs did, in contrast to CLOCK/BMAL1, not strongly activate the circadian reporter genes REVERBα-luc, PER2-luc and SCN5A-luc ( Fig. 1c ). To compare the activating potential of MYC/MAX and CLOCK/BMAL1 at E-boxes we assayed expression of a minimal promoter fused to 6 synthetic E-box elements ( 6xEbox-luc ). Similar synthetic E-box reporters have been shown to be activated by MYC (ref. 15 ). Co-transfection of the 6xEbox-luc reporter with CLOCK and BMAL1 vectors resulted in notably higher luciferase activity than co-transfection with MYC and MAX vectors (14 fold versus 3–4 fold; Fig. 1d ). Interestingly, simultaneous expression of MYC/MAX together with CLOCK/BMAL1 hampered activation of the 6xEbox-luc reporter ( Fig. 1d ). Similarly, MYC/MAX interfered with stronger activation of REVERBα-luc and PER2-luc reporter genes by CLOCK/BMAL1 ( Supplementary Fig. 1b ). The data suggest that MYC/MAX has a weaker activation potential than CLOCK/BMAL1 at synthetic as well as endogenous circadian promoters. Yet, MYC/MAX is functionally dominant over CLOCK/BMAL1. 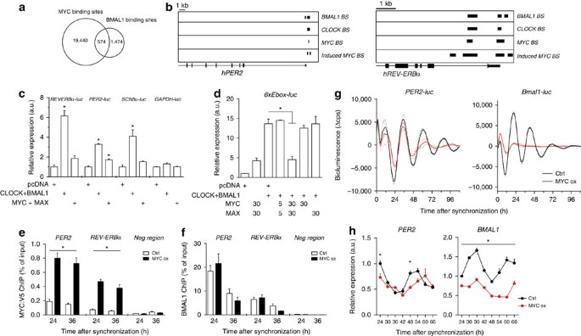Figure 1: Overexpression of MYC attenuates the circadian clock. (a) Overlap between native MYC (ref.14) and BMAL1 (ref.13) binding sites in U2OS cells. (b)PER2andREV-ERBαloci with binding sites (BS) of BMAL1, CLOCK, native MYC and overexpressed MYC in U2OS cells (based on the data from refs13,14). (c) MYC and MAX do not substantially induce the BMAL1/CLOCK target genesREV-ERBα, PER2andSCN5α. HEK293 cells were transfected withMYC,MAX,BMAL1andCLOCKencoding plasmids (30 ng) together with the indicated circadian promoter-luc reporter plasmids.GAPDH-lucwas transfected as a negative control (n=3). (d) MYC/MAX restricts stronger induction of6xEbox-lucby CLOCK/BMAL1. HEK293 cells were transfected with 30 ng of eachBMAL1andCLOCKplasmids, and with the indicated amounts (in ng) ofMYCandMAXvectors (n=3). ChIP-PCR analysis of (e) MYC:V5 and (f) BMAL1 binding to circadian E-boxes inPER2andREV-ERBαpromoters in synchronized and doxycycline-induced U2OSt-rex tetO-MYC:V5cells (n=3). (g) Bioluminescence recorded from synchronizedBmal1-lucandPER2-lucU2OSt-rex tetO-MYC:V5cells (n=3). (h) Quantitative PCR (qPCR) analysis of circadian expression profiles ofPER2andBMAL1transcripts in synchronized U2OSt-rex tetO-MYC:V5cells (n=3). Data are presented as mean±s.e.m. *P<0.05; one-way (c,d) and two-way (e,h) analysis of variance (ANOVA) with Bonferroni post-test. Figure 1: Overexpression of MYC attenuates the circadian clock. ( a ) Overlap between native MYC (ref. 14 ) and BMAL1 (ref. 13 ) binding sites in U2OS cells. ( b ) PER2 and REV-ERBα loci with binding sites (BS) of BMAL1, CLOCK, native MYC and overexpressed MYC in U2OS cells (based on the data from refs 13 , 14 ). ( c ) MYC and MAX do not substantially induce the BMAL1/CLOCK target genes REV-ERBα, PER2 and SCN5α . HEK293 cells were transfected with MYC , MAX , BMAL1 and CLOCK encoding plasmids (30 ng) together with the indicated circadian promoter-luc reporter plasmids. GAPDH-luc was transfected as a negative control ( n =3). ( d ) MYC/MAX restricts stronger induction of 6xEbox-luc by CLOCK/BMAL1. HEK293 cells were transfected with 30 ng of each BMAL1 and CLOCK plasmids, and with the indicated amounts (in ng) of MYC and MAX vectors ( n =3). ChIP-PCR analysis of ( e ) MYC:V5 and ( f ) BMAL1 binding to circadian E-boxes in PER2 and REV-ERBα promoters in synchronized and doxycycline-induced U2OS t-rex tetO-MYC:V5 cells ( n =3). ( g ) Bioluminescence recorded from synchronized Bmal1-luc and PER2-luc U2OS t-rex tetO-MYC:V5 cells ( n =3). ( h ) Quantitative PCR (qPCR) analysis of circadian expression profiles of PER2 and BMAL1 transcripts in synchronized U2OS t-rex tetO-MYC:V5 cells ( n =3). Data are presented as mean±s.e.m. * P <0.05; one-way ( c , d ) and two-way ( e , h ) analysis of variance (ANOVA) with Bonferroni post-test. Full size image Overexpression of MYC disrupts the circadian clock Next, we generated a U2OS cell line expressing a doxycycline-inducible V5-tagged MYC (U2OS t-rex tetO-MYC:V5 ). In presence of doxycycline total MYC (endogenous+induced) was ∼ 9-fold overexpressed ( Fig. 4d and Supplementary Fig. 4c ). Figure 4: MYC mutants compromised in MIZ1 interaction do not disrupt the circadian clock. ( a ) Transactivation assay in HEK293 cells showing that MYC:V5 WT, V394D and V393D equally induce 6xEbox-luc expression and compete with CLOCK/BMAL1 in a dominant negative manner ( n =3). 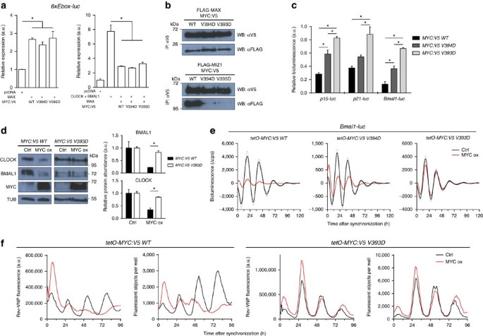Figure 4: MYC mutants compromised in MIZ1 interaction do not disrupt the circadian clock. (a) Transactivation assay in HEK293 cells showing that MYC:V5 WT, V394D and V393D equally induce6xEbox-lucexpression and compete with CLOCK/BMAL1 in a dominant negative manner (n=3). (b) Anti-V5 immunoprecipitation of MYC:V5 versions in HEK293 lysates showing that MYC:V5 V394D and V393D interact with MAX (upper panel) but not with MIZ1 (lower panel). Co-immunoprecipitation (Co-IP) of FLAG-tagged MAX and MIZ1 was detected with anti-FLAG antibodies. Refer toSupplementary Fig. 4afor inputs and reciprocal anti-FLAG co-IP’s. (c) Overexpressed MYC:V5 V394D and V393D are inefficient in repression of MIZ1 target genes. Expression of transiently transfectedp15-luc,p21-lucandBmal1-lucreporters in U2OSt-rex tetO-MYC:V5cells expressing the indicated versions of MYC. Bioluminescence was quantified 18 h after MYC induction with doxycycline and normalized to PBS-treated samples (n=3). (d) Western blot analysis (left) and densitometric protein quantification (right) of CLOCK and BMAL1 in U2OS cells overexpressing MYC and MYC V393D 24 h after doxycycline induction (n=3). (e) Baseline-subtracted bioluminescent traces from U2OSt-rex tetO-MYC:V5 WT,V394DandV393Dcells transiently transfected withBmal1-luc(n=3). For the raw data refer toSupplementary Fig. 4d. (f) Total fluorescence and fluorescent objects quantified from synchronized U2OSt-rex Rev-VNPcells stably transfected with inducibleMYC:V5 WTandV393D(n=1). Data are presented as mean±s.e.m. *P<0.05; one-way analysis of variance (ANOVA) with Bonferroni post-test. ( b ) Anti-V5 immunoprecipitation of MYC:V5 versions in HEK293 lysates showing that MYC:V5 V394D and V393D interact with MAX (upper panel) but not with MIZ1 (lower panel). Co-immunoprecipitation (Co-IP) of FLAG-tagged MAX and MIZ1 was detected with anti-FLAG antibodies. Refer to Supplementary Fig. 4a for inputs and reciprocal anti-FLAG co-IP’s. ( c ) Overexpressed MYC:V5 V394D and V393D are inefficient in repression of MIZ1 target genes. Expression of transiently transfected p15-luc , p21-luc and Bmal1-luc reporters in U2OS t-rex tetO-MYC:V5 cells expressing the indicated versions of MYC. Bioluminescence was quantified 18 h after MYC induction with doxycycline and normalized to PBS-treated samples ( n =3). ( d ) Western blot analysis (left) and densitometric protein quantification (right) of CLOCK and BMAL1 in U2OS cells overexpressing MYC and MYC V393D 24 h after doxycycline induction ( n =3). ( e ) Baseline-subtracted bioluminescent traces from U2OS t-rex tetO-MYC:V5 WT , V394D and V393D cells transiently transfected with Bmal1-luc ( n =3). For the raw data refer to Supplementary Fig. 4d . ( f ) Total fluorescence and fluorescent objects quantified from synchronized U2OS t-rex Rev-VNP cells stably transfected with inducible MYC:V5 WT and V393D ( n =1). Data are presented as mean±s.e.m. * P <0.05; one-way analysis of variance (ANOVA) with Bonferroni post-test. Full size image Twenty four and thirty six hours after induction, MYC:V5 was efficiently recruited to circadian E-box sites in REV-ERBα and PER2 ( Fig. 1e ). Rhythmic recruitment of BMAL1 to these loci was not compromised, yet BMAL1 occupancy was reduced 36 h after induction of MYC:V5 ( Fig. 1f ). The data suggest that at any given time the saturation level of the E-boxes with either transcription factor was rather low such that the transcription factors did not physically compete for common binding sites. The functional dominance of MYC/MAX could reflect a MYC/MAX induced chromatin state that allows binding of CLOCK/BMAL1 but interferes with stronger activation of target genes. We then asked whether overexpression of MYC affects expression levels and circadian rhythms of clock genes. Induction of transgenic MYC:V5 attenuated the circadian expression rhythms of PER2-luc and Bmal1-luc reporters in synchronized U2OS cells, while expression of green fluorescent protein (control) had no effect ( Fig. 1g and Supplementary Fig. 1c,d ). Unexpectedly, however, the expression level and rhythm of the non-E-box-dependent Bmal1-luc reporter were strongly attenuated already shortly after induction of MYC:V5, whereas rhythmic expression of the E-box regulated PER2-luc reporter was affected with delayed kinetics ( Fig. 1g ). Surprisingly, expression levels of PER2-luc decreased in the presence of overexpressed MYC ( Supplementary Fig. 1c ) indicating that the MYC:V5 did not activate the E-box containing circadian promoter. Overexpression of MYC:V5 attenuated expression of endogenous BMAL1 and blunted its circadian profile about 1 day earlier and more strongly than the rhythm of the E-box containing PER2 gene ( Fig. 1g,h ). Furthermore, MYC:V5 expression caused downregulation of the non-E-box genes CLOCK and NPAS2 ( Supplementary Fig. 1e ). It has been suggested that MYC activates REV-ERBα via E-boxes, which in turn would downregulate BMAL1 and thereby attenuate the circadian clock [12] . Indeed, overexpression of a doxycycline-inducible FLAG-tagged REV-ERBα repressed Bmal1-luc levels and damped its rhythms ( Supplementary Fig. 2a ), indicating that REV-ERBα is a potent repressor of BMAL1 in U2OS cells. We therefore asked whether MYC activates REV-ERBα in U2OS cells. Circadian expression profiles revealed that levels of REV-ERBα , as well as of REV-ERBβ , were downregulated rather than activated by overexpressed MYC ( Fig. 2a ). The data are in agreement with the dominant negative effect of MYC/MAX over CLOCK/BMAL1 in transient expression of REVERBα-luc ( Supplementary Fig. 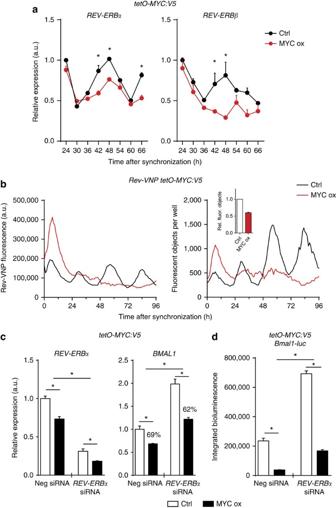1b ). Figure 2: MYC repressesBMAL1independent of REV-ERBα. (a) Quantitative PCR (qPCR) analysis of circadian expression profiles ofREV-ERBαandREV-ERBβtranscripts in synchronized U2OSt-rex tetO-MYC:V5cells (n=3). (b) Total fluorescence and fluorescent objects quantified from synchronized U2OSt-rex Rev-VNP tetO-MYC:V5cells (n=1). Inset: normalized number of fluorescent objects (24–96 h integration;n=2). (c) qPCR analysis ofREV-ERBαandBMAL1transcripts in siRNA-transfected U2OSt-rex tetO-MYC:V5cells (n=3). Unsynchronized cells were collected 24 h after doxycycline induction. (d) Integrated bioluminescence ofBmal1-luctransfected U2OSt-rex tetO-MYC:V5cells. Cells were transfected with indicated siRNAs 2 days before synchronization. Average expression levels (area under the curve) were determined over 72 h (n=3). Data are presented as mean±s.e.m. *P<0.05; two-way analysis of variance (ANOVA) with Bonferroni post-test. Figure 2: MYC represses BMAL1 independent of REV-ERBα. ( a ) Quantitative PCR (qPCR) analysis of circadian expression profiles of REV-ERBα and REV-ERBβ transcripts in synchronized U2OS t-rex tetO-MYC:V5 cells ( n =3). ( b ) Total fluorescence and fluorescent objects quantified from synchronized U2OS t-rex Rev-VNP tetO-MYC:V5 cells ( n =1). Inset: normalized number of fluorescent objects (24–96 h integration; n =2). ( c ) qPCR analysis of REV-ERBα and BMAL1 transcripts in siRNA-transfected U2OS t-rex tetO-MYC:V5 cells ( n =3). Unsynchronized cells were collected 24 h after doxycycline induction. ( d ) Integrated bioluminescence of Bmal1-luc transfected U2OS t-rex tetO-MYC:V5 cells. Cells were transfected with indicated siRNAs 2 days before synchronization. Average expression levels (area under the curve) were determined over 72 h ( n =3). Data are presented as mean±s.e.m. * P <0.05; two-way analysis of variance (ANOVA) with Bonferroni post-test. Full size image To analyse the impact of MYC on REV-ERBα in more detail we constructed a MYC-overexpressing cell line (U2OS t-rex tetO-MYC:V5 ) that expresses under control of the Rev-erbα promoter a destabilized nuclear venus reporter ( Rev-VNP ) [16] . Rev-VNP was rhythmically expressed as assessed by quantifying the total fluorescence and the number of fluorescent objects (cells) per well ( Fig. 2b , black curves). Overexpression of MYC triggered a transient activation of Rev-VNP with a peak ∼ 7 h after induction, which was followed by downregulation and blunting of the circadian Rev-VNP rhythm ( Fig. 2b , red curves). We then integrated over a 3-day time course (24–96 h) the total number of fluorescent objects (cells expressing Rev-VNP above threshold) to assess whether the MYC-dependent loss of rhythmicity in the population of cells was due to desynchronization (same number of fluorescent objects in presence and absence of MYC) or due to an attenuated rhythm, that is, a reduction of the number of highly rhythmic cells (less fluorescent objects above threshold). One day after induction of MYC:V5, the average number of fluorescent objects was ∼ 2-fold reduced, indicating a decrease of the number of highly rhythmic cells rather than desynchronization of the population of cells ( Fig. 2b , inset). MYC-dependent attenuation of the circadian Rev-VNP rhythm rather than MYC-induced desynchronization was also obvious on the level of single cells ( Supplementary Movie 1 ). The data suggest that induction of MYC:V5 does not trigger a sustained overexpression of REV-ERBα but rather reduces its expression level and rhythm. Corresponding results were obtained with a REVERBα-luc reporter ( Supplementary Fig. 2b ). Altman et al . [12] reported induction of REV-ERBα in response to activation of MYC. However, they quantified REV-ERBα at a single time point early after induction of MYC (24 h). At this time REV-ERBα levels may still be slightly elevated due to its transient induction peaking after 7 h ( Fig. 2b ). We thus knocked down REV-ERBα by short interfering RNA (siRNA) to assess whether the MYC-induced downregulation of BMAL1 was dependent on REV-ERBα. REV-ERBα was ∼ 3-fold downregulated by specific versus control siRNA ( Fig. 2c ). When MYC was overexpressed, REV-ERBα levels were additionally reduced by 40% in presence of REV-ERBα specific siRNA and by 25% in presence of control siRNA ( Fig. 2c ). Downregulation of REV-ERBα by siRNA resulted in elevated expression of BMAL1 ( Fig. 2c ), indicating that REV-ERBα is a potent repressor of BMAL1 in U2OS cells. However, overexpressed MYC repressed BMAL1 in both, REV-ERBα depleted and control cells (62 and 69%, respectively), indicating that MYC acted independent of REV-ERBα . Corresponding results were obtained with a Bmal1-luc reporter ( Fig. 2d ). Downregulation of the positive limb of the circadian feedback loop has been shown to be sufficient to disrupt the molecular clock in U2OS cells [17] . Accordingly, the MYC-dependent attenuation of expression level and circadian rhythm of Bmal1-luc was partially rescued by constitutive overexpression of BMAL1 together with CLOCK ( Supplementary Fig. 2c,d ). Together, these data suggest that overexpression of MYC did not enhance expression of REV-ERBα in a sustained manner. Rather, overexpressed MYC compromised the circadian system primarily via downregulation of BMAL1 , CLOCK and its homologue NPAS2 by a pathway independent of REV-ERBα and REV-ERBβ. MYC represses the circadian clock via interaction with MIZ1 MYC is not only a transcription activator. When expressed at high level, MYC has the potential to form a repressive complex with MIZ1 (ZBTB17) and downregulate in E-box-independent fashion expression of MIZ1 target genes such as the cyclin-dependent kinase inhibitor genes p15 and p21 (refs 14 , 18 , 19 ). We followed the MYC-dependent temporal expression profiles of luciferase reporter constructs of established and putative MIZ1 target genes. After induction of MYC:V5 with doxycycline, Bmal1-luc was repressed with similar kinetics as p15-luc and p21-luc , while 6xEbox-luc was, as expected, induced when MYC was overexpressed ( Fig. 3a ). Examining a published ChIP-seq analysis of MIZ1 in U2OS cells [14] , we realized that MIZ1 binds to the promoters of BMAL1, CLOCK and NPAS2 ( Fig. 3b , left panel). We therefore performed a ChIP-PCR analysis and found that overexpressed MYC:V5 was recruited to the MIZ1 sites in BMAL1 , CLOCK and NPAS2 ( Fig. 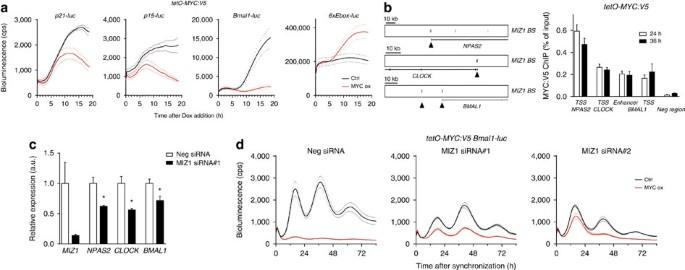3b , right panel), suggesting that MYC binds to and represses these genes via MIZ1. Figure 3: MYC directly represses clock genes via MIZ1. (a) Kinetics of MYC-dependent repression ofp21-luc,p15-lucandBmal1-lucand activation of6xEbox-luc(n=3). Unsynchronized U2OSt-rex tetO-MYC:V5cells were transiently transfected with the indicated reporter plasmids. At time point 0 MYC:V5 expression was either induced with doxycycline (MYC ox) or not induced with PBS (Ctrl). (b) Left panel: schematic of MIZ1 binding sites inNPAS2,CLOCKandBMAL1based on data from Walzet al.14. Black triangles indicate regions amplified in ChIP-PCR analysis. Right panel: ChIP-PCR analysis showing recruitment of induced MYC:V5 to MIZ1 binding sites inNPAS2,CLOCKandBMAL1at 24 and 36 h after synchronization of U2OSt-rex tetO-MYC:V5cells (n=3). (c) Downregulation ofMIZ1with siRNA reduces expression ofNPAS2,CLOCKandBMAL1in U2OS cells (n=3). Transcript levels of the indicated genes were determined by quantitative PCR (qPCR). (d) MYC-induced attenuation of the circadian clock is rescued by downregulation of MIZ1 (n=3). Synchronized U2OSt-rex tetO-MYC:V5 Bmal1-luccells were transfected withMIZ1or control siRNAs. Note that downregulation ofMIZ1attenuates the circadian rhythm ofBmal1-lucand lengthens the period (Supplementary Fig. 3a,b). Data are presented as mean±s.e.m. *P<0.05; Student’st-test. Figure 3: MYC directly represses clock genes via MIZ1. ( a ) Kinetics of MYC-dependent repression of p21-luc , p15-luc and Bmal1-luc and activation of 6xEbox-luc ( n =3). Unsynchronized U2OS t-rex tetO-MYC:V5 cells were transiently transfected with the indicated reporter plasmids. At time point 0 MYC:V5 expression was either induced with doxycycline (MYC ox) or not induced with PBS (Ctrl). ( b ) Left panel: schematic of MIZ1 binding sites in NPAS2 , CLOCK and BMAL1 based on data from Walz et al . [14] . Black triangles indicate regions amplified in ChIP-PCR analysis. Right panel: ChIP-PCR analysis showing recruitment of induced MYC:V5 to MIZ1 binding sites in NPAS2 , CLOCK and BMAL1 at 24 and 36 h after synchronization of U2OS t-rex tetO-MYC:V5 cells ( n =3). ( c ) Downregulation of MIZ1 with siRNA reduces expression of NPAS2 , CLOCK and BMAL1 in U2OS cells ( n =3). Transcript levels of the indicated genes were determined by quantitative PCR (qPCR). ( d ) MYC-induced attenuation of the circadian clock is rescued by downregulation of MIZ1 ( n =3). Synchronized U2OS t-rex tetO-MYC:V5 Bmal1-luc cells were transfected with MIZ1 or control siRNAs. Note that downregulation of MIZ1 attenuates the circadian rhythm of Bmal1-luc and lengthens the period ( Supplementary Fig. 3a,b ). Data are presented as mean±s.e.m. * P <0.05; Student’s t -test. Full size image When MYC is not overexpressed MIZ1 acts as a transcription activator [20] . To assess whether MIZ1 supports expression of BMAL1 , CLOCK and NPAS2 in U2OS cells, we depleted MIZ1 with siRNA ( Fig. 3c ). Expression of BMAL1 , CLOCK and NPAS2 was reduced indicating that MIZ1 contributes to the transcriptional activation of these clock genes. When MIZ1 was depleted by siRNAs, the circadian expression rhythm of Bmal1-luc was weakened in comparison to a treatment with control siRNA ( Fig. 3d , black curves) and the circadian period was lengthened ( Supplementary Fig. 3a ). To assess whether the MYC-dependent disruption of the clock requires MIZ1, we induced MYC:V5 in MIZ1-depleted and control-treated cells ( Fig. 3d , red curves). As expected, the circadian expression rhythm of Bmal1-luc was abolished when MYC:V5 was overexpressed in control-treated cells ( Fig. 3d , red curve left panel). Concomitant downregulation of MIZ1, however, partially restored the expression level and circadian rhythms of Bmal1-luc despite overexpression of MYC:V5 ( Fig. 3d , red curves middle and right panels). Correspondingly, the rhythm of 6xEbox-luc was severely attenuated by induced MYC:V5 and fully rescued by siRNA depletion of MIZ1 ( Supplementary Fig 3b ). Together the data indicate that overexpressed MYC represses BMAL1 directly via MIZ1-dependent recruitment of MYC to MIZ1 binding sites. MYC-mediated attenuation of the clock requires MIZ1 To challenge this hypothesis, we generated the V5-tagged MYC V394D mutant, which is impaired in its interaction with MIZ1 (ref. 21 ) and in addition the variant V393D. ChIP-PCR analysis demonstrated that, as was shown for V394D [21] , the newly generated V393D variant binds with similar affinity to E-boxes as WT MYC ( Supplementary Fig. 4a ). Both mutant versions of MYC:V5 induced expression of 6xEbox-luc in HEK293 cells and interfered in dominant negative fashion with CLOCK/BMAL1-dependent activation of 6xEbox-luc to the same extent as wild-type MYC:V5 ( Fig. 4a ). Theses data suggest that the E-box-dependent functionality of MYC:V5 V394D and MYC:V5 V393D was not affected. Both mutant versions interacted with MAX with similar efficiency as MYC:V5 ( Fig. 4b , upper panel; and Supplementary Fig. 4b ). In contrast, the V394D and V393D variants showed markedly reduced association with MIZ1 ( Fig. 4b , lower panel; and Supplementary Fig. 4b ). Next, we produced stable U2OS cell lines harbouring doxycycline-inducible MYC:V5 V394D and MYC:V5 V393D genes. Both inducible transcripts accumulated to similar levels as MYC:V5 ( Supplementary Fig. 4c ). However, repression of p15-luc, p21-luc as well as Bmal1-luc reporters was alleviated in the cell lines expressing the V393D and V394D versions of MYC:V5 ( Fig. 4c ). The levels of CLOCK and BMAL1 proteins were strongly reduced by overexpression of MYC:V5, but remained essentially unaffected by induction of MYC:V5 V393D ( Fig. 4d ). Circadian expression rhythms of Bmal1-luc and 6xEbox-luc reporters were strongly attenuated by overexpression of wild-type MYC:V5, but only mildly affected by overexpression of V394D and essentially unaffected by the V393D version ( Fig. 4e and Supplementary Fig. 4d ). Similarly, Rev-VNP (ref. 16 ) expression levels and rhythms were strongly attenuated by overexpressed MYC:V5 but unaffected by induction of MYC:V5 V393D ( Fig. 4f and Supplementary Movies 1 and 2 ). The data demonstrate that overexpressed MYC attenuates the circadian clock via MIZ1-mediated E-box-independent repression. MYC-dependent cell cycle stimulation requires MIZ1 Elevated MYC expression is considered to drive cell growth and proliferation through genome-wide interference with physiological regulation of E-box-dependent transcription [22] . Since the E-box-dependent activation properties are preserved in the V393D version of MYC:V5 ( Fig. 4a ), we asked how it affects cell growth and proliferation. Consistent with previous studies [21] , induction of MYC:V5 reduced the fraction of cells in G1 phase and increased the proportion of cells in S, G2 and M phases ( Fig. 5a,b ). In contrast, overexpression of MYC:V5 V393D did not support proliferation to a substantial extent. These data suggest that stimulation of proliferation of U2OS cells by MYC is crucially dependent on gene repression via MIZ1. Together the data suggest that overexpression of MYC supports proliferation and attenuates the circadian clock predominantly via MIZ1. 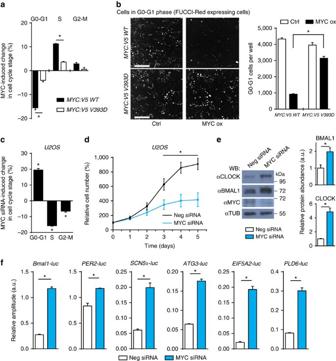Figure 5: MYC inversely regulates the circadian clock and proliferation. (a)MYC:V5 WTandV393DU2OS cells were stained with propidium iodide 48 h after induction and DNA content was quantified by FACS (n=3). Values indicate difference (in %) to PBS-treated cells in the respective cell cycle phase. (b) Left panel: fluorescence microscopy of U2OSt-rex tetO-MYC:V5cells stably expressing mCherry-Cdt1 (FUCCI-Red G1 marker) 48 h after treatment with doxycycline to induce MYC:V5 (MYC ox) or PBS (Ctrl). Scale bar, 300 μm. Right panel: quantification of cells in G0 or G1 phase by mCherry-Cdt1 expression (n=3) (c) FACS analysis of U2OS cells stained with propidium iodide 48 h after transfection with MYC siRNA (n=3). Values indicate difference to cells transfected with negative siRNA. (d) Growth curve of U2OS cells transfected with MYC siRNA and negative siRNA (n=3). (e) Western blot analysis (left) and densitometric protein quantification (right) showing that MYC depletion by siRNA supports increased BMAL1 and CLOCK expression in U2OS cells (n=3). (f) Relative amplitudes (ChronoStar software) of circadian luciferase rhythms of indicated U2OS reporter cell lines (n=3). The cells were transfected with MYC siRNA and negative siRNA as indicated. Data are presented as mean±s.e.m. *P<0.05; Student’st-test (e,f), one-way (b,c) and two-way (a,d) analysis of variance (ANOVA) with Bonferroni post-test. Figure 5: MYC inversely regulates the circadian clock and proliferation. ( a ) MYC:V5 WT and V393D U2OS cells were stained with propidium iodide 48 h after induction and DNA content was quantified by FACS ( n =3). Values indicate difference (in %) to PBS-treated cells in the respective cell cycle phase. ( b ) Left panel: fluorescence microscopy of U2OS t-rex tetO - MYC:V5 cells stably expressing mCherry-Cdt1 (FUCCI-Red G1 marker) 48 h after treatment with doxycycline to induce MYC:V5 (MYC ox) or PBS (Ctrl). Scale bar, 300 μm. Right panel: quantification of cells in G0 or G1 phase by mCherry-Cdt1 expression ( n =3) ( c ) FACS analysis of U2OS cells stained with propidium iodide 48 h after transfection with MYC siRNA ( n =3). Values indicate difference to cells transfected with negative siRNA. ( d ) Growth curve of U2OS cells transfected with MYC siRNA and negative siRNA ( n =3). ( e ) Western blot analysis (left) and densitometric protein quantification (right) showing that MYC depletion by siRNA supports increased BMAL1 and CLOCK expression in U2OS cells ( n =3). ( f ) Relative amplitudes (ChronoStar software) of circadian luciferase rhythms of indicated U2OS reporter cell lines ( n =3). The cells were transfected with MYC siRNA and negative siRNA as indicated. Data are presented as mean±s.e.m. * P <0.05; Student’s t -test ( e,f ), one-way ( b , c ) and two-way ( a , d ) analysis of variance (ANOVA) with Bonferroni post-test. Full size image Knockdown of MYC induces circadian amplitude Next, we analysed effects of MYC depletion. Knockdown of MYC by siRNA resulted in decreased proliferation of U2OS cells ( Fig. 5c,d ). Concomitantly, expression levels of BMAL1 and CLOCK increased ( Fig. 5e ). Furthermore, the relative amplitudes (the oscillation amplitude divided by the mean expression) of the circadian expression rhythms of Bmal1-luc and other circadian reporters significantly improved in cells transfected with MYC siRNA ( Fig. 5f and Supplementary Fig. 5a ). Corresponding effects were observed in U2OS cells expressing Rev-VNP ( Supplementary Fig. 5b , Supplementary Movie 3 ). Thus, downregulation of MYC with siRNA increased the relative amplitude of the Rev-VNP rhythm. In summary, the data indicate that downregulation of MYC attenuates proliferation and strengthens the circadian clock. Inverse correlation of MYC and clock genes in lymphoma MYC is overexpressed in many tumours and depletion of MYC is known to detain tumour growth [22] . Encouraged by the inverse correlation of MYC with BMAL1 and CLOCK expression in U2OS cells, we assessed expression of these genes in human lymphoma by analysing RNA-seq data of 102 patient samples. Lymphoma was chosen since this type of malignancy requires interaction of MYC and MIZ1 (ref. 23 ). Consistent with our observation in U2OS cells, expression of both clock genes correlated inversely with MYC levels in human lymphoma (Pearson coefficient −0.61 and −0.37 for BMAL1 and CLOCK , respectively; n =102), whereas MYC-activated genes such as NCL and NCLN showed a positive correlation ( Fig. 6a,b and Supplementary Fig. 6 ). MYC levels did not correlate positively with expression of circadian genes regulated via E-boxes. Particularly, REV-ERBα and β did not significantly correlate with MYC . 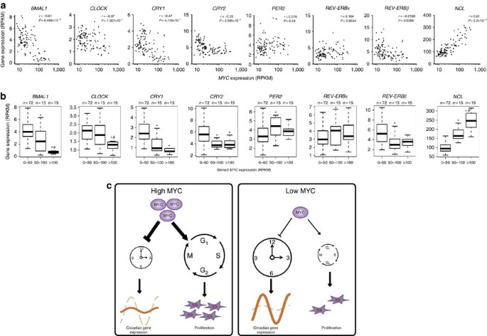Figure 6:MYCinversely correlates withBMAL1expression in human lymphomas. (a) Scatter plots of expression levels ofMYCversus the indicated clock genes in 102 human lymphoma samples of the ICGC MMML-Seq project37(RPKM: log2 sequence reads per kilobase transcript per million reads38). Expression ofMYCversus its established targetNUCLEOLIN(NCL) is shown as a positive control. (b) Data were binned according to the indicated MYC expression levels. Clock gene expression levels are shown by Box-plots. Significant differences (P<0.05; Student’st-test) of expression levels relative to box 1 (0–50) and box 2 (50–100) are indicated by asterisks (*) and number signs (#), respectively. (c) Model of the coordinating function of MYC. Left panel: high levels of MYC suppress the circadian clock by MIZ1-dependent downregulation of BMAL1/CLOCK (see text), which results in low amplitude expression rhythms of clock-controlled genes. On the other hand, high MYC levels support cell growth and proliferation (for example, by inhibition ofp15andp21, see text). Right panel: at low levels of MYC, the circadian clock is not inhibited and supports high amplitude expression rhythms of clock-controlled genes. Low levels of MYC do not support cell growth and proliferation. Figure 6: MYC inversely correlates with BMAL1 expression in human lymphomas. ( a ) Scatter plots of expression levels of MYC versus the indicated clock genes in 102 human lymphoma samples of the ICGC MMML-Seq project [37] (RPKM: log2 sequence reads per kilobase transcript per million reads [38] ). Expression of MYC versus its established target NUCLEOLIN ( NCL ) is shown as a positive control. ( b ) Data were binned according to the indicated MYC expression levels. Clock gene expression levels are shown by Box-plots. Significant differences ( P <0.05; Student’s t -test) of expression levels relative to box 1 (0–50) and box 2 (50–100) are indicated by asterisks (*) and number signs (#), respectively. ( c ) Model of the coordinating function of MYC. Left panel: high levels of MYC suppress the circadian clock by MIZ1-dependent downregulation of BMAL1/CLOCK (see text), which results in low amplitude expression rhythms of clock-controlled genes. On the other hand, high MYC levels support cell growth and proliferation (for example, by inhibition of p15 and p21 , see text). Right panel: at low levels of MYC, the circadian clock is not inhibited and supports high amplitude expression rhythms of clock-controlled genes. Low levels of MYC do not support cell growth and proliferation. Full size image The circadian clock and cell cycle/proliferation are major programs controlling expression of specific, potentially overlapping sets of genes [24] , [25] , [26] , [27] . Since the simultaneous regulatory activity of both programs in the same cell may create conflicting signals, it seems conceivable that their activity is coordinated under physiological conditions. It has been shown that in regenerating mouse liver, the circadian clock gates the cell cycle [28] and that in NIH3T3 cells the cell cycle resets the circadian clock [29] , [30] . The circadian clock in the liver of a living animal oscillates with high amplitude, while the circadian clock in isolated cells appears to be substantially weaker [13] , [31] . Hence, the dominance of one cycling programme over the other may depend on their relative strength or rhythmic momentum. Our observations suggest that MYC is a master regulator coordinating both programs. Expression levels of MYC determine the relative strength of the circadian clock versus cell cycle/proliferation and hence, their impact on gene expression and cellular physiology. MYC attenuates the circadian system and promotes proliferation. Both functions are critically dependent on complexes of MYC with MIZ1. Such repressive complexes form preferentially at high MYC levels [32] . The inverse correlation of BMAL1 versus MYC expression levels in human lymphomas and the absence of a positive correlation of MYC with circadian E-box genes support this hypothesis. The correlation suggests that circadian physiology might be compromised in tumours with amplified MYC . Strategies targeting the interaction of MYC with MIZ1 could help to recover circadian control over cellular physiology in malignant cells and potentially inhibit uncontrolled growth without major effects on differentiated post-mitotic cells with low MYC expression. It seems conceivable that rhythmic downregulation of metabolic and biosynthetic functions by the circadian clock may be in conflict with rapid cell growth and proliferation. Hence, aside from malignant conditions, MYC may also coordinate the relative impact on gene expression of the circadian clock versus cell cycle/proliferation under physiological conditions such as in the developing and differentiating embryo. Cell culture and transfections U2OS t-rex (T-Rex, Life Technologies) and HEK293T (ATCC) cells were maintained in DMEM supplemented with 10% fetal bovine serum (FBS) and 1xPenStrep. Cell culture reagents were obtained from Life Technologies unless indicated differently. U2OStx were transfected with AhdI -linearized pcDNA4/TO vectors containing different alleles of human MYC using Xfect (Clontech) and stable transfectants were selected using growth medium supplemented with 50 μg ml −1 hygromycin and 100 μg ml −1 zeocin (InvivoGen). Positive clones were subsequently, transiently or stably transfected with circadian reporter constructs using Xfect reagent and, if applicable, selected with 1 μg ml −1 puromycin (InvivoGen). U2OS stable cell lines expressing the promoter-luciferase constructs were described previously [13] . For RNAi experiments, U2OS cells were transfected with the indicated siRNA (sequences are given in Supplementary Table 1 ) using lipofectamine RNAiMAX reagent according to manufacturer’s protocols. For luciferase reporter assays, HEK293T cells were transfected with the indicated constructs using Lipofectamine2000 and 24 h later luciferase expression was assayed using Dual-luciferase Reporter Assay (Promega) and an EnSpire Reader (Perkin Elmer). Plasmid constructs Bmal1-luc and 6xEbox-luc vectors were kindly provided by Dr Steven A Brown and Dr Achim Kramer [33] , [34] . p15-luc , p21-luc and MIZ1 open reading frame (ORF) vectors were kindly provided by Dr Elmar Wolf. Rev-VNP fluorescent reporter containing 13 kb of murine Rev-erbα promoter coupled to Venus-NLS-PEST was kindly provided by Dr Ueli Schibler. Promoter sequences (1 kb) of PER2, REV-ERBα, SCN5α and GAPDH genes cloned in pGL4.20puro vector were described previously [13] . BMAL1 , CLOCK and MAX ORFs were amplified from U2OS complementary DNA (cDNA) and cloned in pcDNA4/TO vector. The MYC and FLAG:REV-ERBα ORFs were obtained from Addgene and subcloned in pcDNA4/TO. MYC V394D and V393D mutations were performed using DF-Pfu polymerase (Bioron). Cloning and mutagenesis primers are available on request. Real-time bioluminescence monitoring For RNAi or transfection experiments, cells were seeded into a 96-well plate (20,000–30,000 cells per well) and next day transfected with the indicated siRNAs. 24 h later the transfection medium was removed and cells were synchronized with 1 μM dexamethasone for 20 min and washed with PBS. After addition of warm luminescene medium (DMEM w/o Phenolred (PAA) supplemented with 10% FBS, 25 mM Hepes, 1xPenStrep, and 0.125 μM luciferin (BioSynth), 10ng ml −1 doxycycline) the plate was sealed and bioluminescence was recorded for 30 min intervals at 37 °C with an EnSpire Reader (Perkin Elmer). Circadian period and amplitude analysis was performed using ChronoStar software [35] . Gene expression analysis Transfected or synchronized cells were lysed with TriFaster (GeneON) and total RNA was extracted according to manufacturer’s protocol. cDNA was synthesized with Maxima First Strand cDNA Synthesis Kit (Thermo Scientific). Quantitative PCR was performed using GoTaq Master Mix (Promega) and LightCycler 480 (Roche) and relative gene expression was quantified using a ΔΔCt method with GAPDH as a reference gene. Primer sequences are listed in Supplementary Table 1 . Chromatin immunoprecipitation (ChIP) U2OS t-rex cells were collected 24 and 36 h after synchronization (10 ng ml −1 doxycycline added at time point 0) and immediately cross-linked in 1% formaldehyde for 10 min. ChIP was performed as described previously with minor modifications [36] . In brief, pelleted nuclei were suspended in 300 μl IP buffer (150 mM NaCl, 5 mM EDTA, NP-40 (0.5%), Triton X100 (1.0%), 50 mM Tris-HCl, pH 7.5) supplemented with 0.1% SDS and sonicated (30 s on/30 s off cycles for 20 min) using a Bioruptor (Diagenode Inc.). Sheared chromatin (equivalent of 10 6 cells) was incubated overnight at 4 °C with 3 μl of anti-BMAL1 (ref. 13 ; 0.1 mg ml −1 ) and 0.5 μl anti-V5 antibodies (1 mg ml −1 , 46-0705, Life Technologies), and obtained immune complexes were precipitated with salmon sperm DNA blocked protein A-agarose beads (Millipore) equilibrated five times with IP buffer. Precipitated DNA was recovered by boiling for 10 min in 10% Chelex slurry (Bio-Rad) followed by Proteinase K (150 μg ml −1 , New England Biolabs) treatment at 55 °C for 30 min. Proteinase K was subsequently inhibited by boiling at 95 °C for 10 min and beads were removed by centrifugation at 12,000 g at 4 °C. DNA-containing supernatants were analysed by quantitative PCR, and values were normalized to percentage of input. Primer sequences are listed in Supplementary Table 1 . Cell proliferation assays Prior to siRNA transfection, U2OS t-rex cells were seeded on 96-well plates (5,000 cells per well) in 100 μl DMEM (10% FBS, 1xPenStrep). Twenty four hours after transfection (day 0), medium was replaced with 100 μl DMEM (10% FBS, 1xPenStrep). Cell number was measured daily by incubating cells for 1.5 h with DMEM containing 1/10 diluted WST-8 reagent at 37 °C (Cell Counting Kit-8, Sigma-Aldrich) and absorbance was read at 450 nm using an EnSpire Reader (Perkin Elmer). Fluorescent microscopy U2OS t-rex Rev-VNP ( tetO-MYC WT/V393D or siRNA transfected) cells were seeded (10,000 cells per well) on ImageLock 96-well plates (Essen Bioscience) in 100 μl DMEM (10% FBS, 1xPenStrep). Next day, after dexamethasone synchronization and PBS wash, cells were incubated in 100 μl PBS- or Doxycycline-containing DMEM (10% FBS, 1xPenStrep) and monitored with IncuCyte ZOOM reader (Essen Bioscience). To detect cells in G0–G1 phase, U2OS overexpressing MYC alleles were stably transfected with FUCCI-Red construct and puromycin-resistant clones were selected. Then 7,000 cells were seeded on ImageLock 96-well plates (Essen Bioscience) and next day, after addition of doxycycline, cells were monitored with an IncuCyte ZOOM reader (Essen Bioscience) and red-fluorescent objects were counted using in-built software. Total fluorescence and number of fluorescent objects were measured using in-built software. FACS After 3 days of doxycycline induction, trypsinized and PBS-washed cells ( ∼ 10 6 cells) were fixed in 70% ethanol for 1 h at 4 °C. After centrifugation for 5 min at 300 g , cells were washed once with PBS and incubated for 10 min at room temperature in 1 ml propidium iodide-staining solution (PBS, 0.1% TritonX-100, 10 μg ml −1 freshly added propidium iodide, 100 μg ml −1 freshly added RNaseA). Cellular DNA content was measured with a FACSCanto analyzer (BD). Co-immunoprecipitation (Co-IP) and western blotting For protein analysis, synchronized U2OS cells were lysed in ice-cold lysis buffer (25 mM Tris-HCl, pH 8.0, 150 mM NaCl, 0.5% Triton X100, 2 mM EDTA, 1 mM NaF and protease inhibitor cocktail (Roche, 04693159001)) for 10 min on ice and sonicated in ice water in an ultrasonic bath (Merck) for 10 min. Then lysates were pre-cleared from cell debris by centrifugation at 16,000 g for 15 min at 4 °C and the protein concentration in the supernatant was determined with Roti-Quant (Carl Roth). Samples (200 μg of total protein) were boiled with the appropriate amount of 4x Laemmli buffer (250 mM Tris-HCl pH 6.8, 6% SDS, 40% Glycerol, 0.04% Bromphenolblue and 20% Mercaptoethanol) for 3 min at 95 °C and separated using 12% SDS-PAGE. After semi-dry transfer (PEQLAB) on nitrocellulose membranes (GE Healthcare), protein extracts were decorated with anti-BMAL1 (ref. 13 ; 1:750), anti-CLOCK (ref. 13 ; 1:500), anti-MYC (1:400, N-262, SantaCruz), anti-V5 (1:5,000, 46-0705, Life Technologies) and anti-FLAG (1:5,000, M2, Sigma-Aldrich) antibodies in 5% milk TBS at 4 °C overnight. Next day, membrane was washed three times in TBS and incubated with the appropriate HRP-conjugated secondary antibody in 5% milk TBS for 1 h at room temperature. After 4 TBS washes, the membrane was exposed to X-ray films (Super RX, FUJIFILM) and developed using an AGFA automatic processor developer. For co-IP, lysates from transfected HEK293T cells were prepared as described above. Lysates (500 μg total protein) were incubated with anti-V5 (0.5 μl) antibodies or 40 μl of PBS-washed anti-FLAG M2 Affinity Gel (Sigma-Aldrich) agitating at 4 °C overnight. Next day, 40 μl of PBS-washed protein A sepharose beads (GE Healthcare) were added to bind anti-V5 immune complexes and incubated for 2 h. Then beads were washed three times with PBS and protein was eluted by boiling in 4x Laemmli buffer. Precipitated proteins were analysed by western blotting as described above. Uncropped blots are shown in Supplementary Fig. 7 . How to cite this article: Shostak, A. et al . MYC/MIZ1-dependent gene repression inversely coordinates the circadian clock with cell cycle and proliferation. Nat. Commun. 7:11807 doi: 10.1038/ncomms11807 (2016).